Tumour PDGF-BB expression levels determine dual effects of anti-PDGF drugs on vascular remodelling and metastasis Anti-platelet-derived growth factor (PDGF) drugs are routinely used in front-line therapy for the treatment of various cancers, but the molecular mechanism underlying their dose-dependent impact on vascular remodelling remains poorly understood. Here we show that anti-PDGF drugs significantly inhibit tumour growth and metastasis in high PDGF-BB-producing tumours by preventing pericyte loss and vascular permeability, whereas they promote tumour cell dissemination and metastasis in PDGF-BB-low-producing or PDGF-BB-negative tumours by ablating pericytes from tumour vessels. We show that this opposing effect is due to PDGF-β signalling in pericytes. Persistent exposure of pericytes to PDGF-BB markedly downregulates PDGF-β and inactivation of the PDGF-β signalling decreases integrin α1β1 levels, which impairs pericyte adhesion to extracellular matrix components in blood vessels. Our data suggest that tumour PDGF-BB levels may serve as a biomarker for selection of tumour-bearing hosts for anti-PDGF therapy and unsupervised use of anti-PDGF drugs could potentially promote tumour invasion and metastasis. The platelet-derived growth factor (PDGF) family consists of four structurally related members, PDGF-A, -B, -C and -D [1] , [2] . These ligands bind with high specificity to two cell membrane tyrosine kinases, PDGF receptor (PDGFR)-α and -β, that interact to form three dimeric receptor isoforms, PDGFR-αα, -ββ, and -αβ. PDGF-BB is a pluripotent angiogenic ligand; it activates all three receptor isoforms to induce target cell proliferation, migration and survival [3] , [4] , [5] , [6] , [7] , [8] , [9] , [10] , [11] , [12] , [13] , [14] , [15] . In mice, genetic deletion of PDGF-BB or PDGFR-β results in a series of vascular abnormalities in association with pericyte loss including vessel dilation, leakage and rupture, and irregular vascular networks. These abnormalities lead to lethal haemorrhage and oedema in early embryonic development [16] , [17] . Pericyte deficiency-related vascular abnormalities resemble those found in tumours, suggesting that pericyte loss significantly contributes to the tortuosity of tumour vascular networks [18] , [19] . Endothelial cell (EC)-derived PDGF-BB mediates recruitment of pericytes to angiogenic vessels [17] , [20] . However, the relation between PDGF-BB-producing cell types and vascular abnormalities in the tumour environment has poorly been studied. The function of vascular pericytes in tumour growth, metastasis, and responsiveness to antiangiogenic drugs also remains unclear. Particularly, various tumours produce different levels of PDGF-BB, which may result in opposing effects on pericyte coverage or repelling in angiogenic vessels. In the view of variation of vascular remodelling promoted by different levels of PDGF-BB, the anti-PDGF drugs may produce diverse beneficial effects in cancer patients. We demonstrate that tumour-derived PDGF-BB above a threshold level significantly ablates pericytes from the tumour microvasculature via activation of the PDGFR-β-signalling pathway. These findings are clinically relevant in the light of existence of similar PDGF-BB levels in certain human tumours. Furthermore, PDGF-BB-induced pericyte loss, vascular permeability and disorganized vascular architecture lead to enhanced metastatic potentials by increasing dissemination of malignant cells into the circulation. Based on these findings, it is reasonable to speculate that inhibition of the PDGF-BB/PDGFR-β signalling in high PDGF-BB-expressing tumours would be beneficial for cancer therapy. Paradoxically, in low PDGF-producing tumours PDGF blockades would probably further increase the vascular leakiness by ablating pericytes from tumour vessels, leading to potentially increased tumour invasion. Pericyte loss in PDGF-BB-producing human tumours We analysed PDGF-BB in the conditioned medium secreted by a range of human tumour cell lines and correlated the tumour cell PDGF-BB production with pericyte ablation. These cell lines included A431 vulva epidermoid carcinoma, A549 lung adenocarcinoma, ACHN and CAKI-1 renal cell carcinoma, IMR32 neuroblastoma, MDA-MB 231 and MCF7 breast adenocarcinoma, OVCAR4 and OVCAR8 ovarian adenocarcinoma, and U251 glioblastoma. Among these human tumour cell lines, A431 expressed the highest level of PDGF-BB as measured in vivo tumour tissues, whereas other tumour tissues expressed relatively lower PDGF-BB protein. We chose A431 and IMR32 as PDGF-BB-high and -low-expressing tumours for vascular analysis ( Fig. 1a ). Intriguingly, the total number of NG2, the pericyte-specific proteoglycan, positive pericytes was markedly lesser in high PDGF-BB-producing A431 tumours than that in low PDGF-BB-expressing IMR32 tumours ( Fig. 1b ). Pericyte coverage was significantly reduced and a substantial number of residual pericytes remained disassociated from tumour vessels in A431 tumours ( Fig. 1b ). These surprising findings suggest that high levels of PDGF-BB might contribute to pericyte loss in tumour tissues. 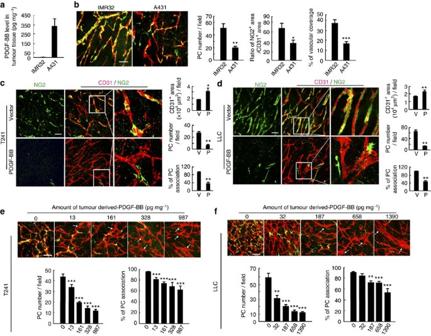Figure 1: PDGF-BB-induced dose-dependent vascular effects in tumours. (a) PDGF-BB expression levels detected by ELISA in human A431 and IMR32 tumour tissues. (b) Left: Representative images of tumour microvasculatures and pericyte coverage in human tumours detected using anti-CD31 (red) and anti-NG2 (green) double immunostaining. Green colour indicates vasculature-disassociated pericytes. Right: Quantification of pericyte numbers in tumours (n=7 fields per group), the ratio of NG2+pericyte versus CD31+microvessels (n=7 fields per group) and pericyte coverage in tumour vasculatures (n=7 fields per group). (c) Left: T241-vector and -PDGF-BB tumour tissues were double immunostained using anti-CD31 (red) and anti-NG2 (green). Yellow colour=vasculature-associated pericytes; green colour=pericytes-disassociated from the tumour vasculature. The right panels reflect magnification of the boxed regions in the middle panels ( × 20). Right: Quantification of microvasculature areas (top) (n=7–9), pericyte numbers (middle) (n=7), pericyte association (bottom) (n=7) in T241-vector and -PDGF-BB tumours. (d) Left: LLC-vector and -PDGF-BB tumour tissues were immunostained as ina. Yellow colour=vasculature-associated pericytes; green colour=pericytes disassociated from the tumour vasculature. Right: Quantification of microvasculature areas (top) (n=7–9), pericyte numbers (middle) (n=7), pericyte association (bottom) (n=7) in LLC-vector and -PDGF-BB tumours. (e,f) Top: T241-vector and -PDGF-BB (c) or LLC-vector and -PDGF-BB (d) tumour cells were mixed at different ratios and implanted in C57Bl/6 mice. The tumour vasculature and pericyte association were detected using anti-CD31 (red) and anti-NG2 (green) double immunostaining. Expression levels of PDGF-BB in tumours were analysed by ELISA. Yellow colour indicates vasculature-associated pericytes and green colour indicates pericytes disassociated from the vasculature. Arrows ine,findicate the dilated and disorganized tumour vasculatures. Bottom: Quantification of pericyte numbers in vector and PDGF-BB tumours (n=7) and pericyte association in control and PDGF-B tumour vasculatures (n=7). All quantifications were performed using the × 20 magnification. Scale bar, 50 μm (in all images); V, vector tumours; P, PDGF-BB tumours. All data are repeated at least twice and represented as mean±s.e.m. *P<0.05; **P<0.01; ***P<0.001 (Student’st-test). Figure 1: PDGF-BB-induced dose-dependent vascular effects in tumours. ( a ) PDGF-BB expression levels detected by ELISA in human A431 and IMR32 tumour tissues. ( b ) Left: Representative images of tumour microvasculatures and pericyte coverage in human tumours detected using anti-CD31 (red) and anti-NG2 (green) double immunostaining. Green colour indicates vasculature-disassociated pericytes. Right: Quantification of pericyte numbers in tumours ( n =7 fields per group), the ratio of NG2 + pericyte versus CD31 + microvessels ( n =7 fields per group) and pericyte coverage in tumour vasculatures ( n =7 fields per group). ( c ) Left: T241-vector and -PDGF-BB tumour tissues were double immunostained using anti-CD31 (red) and anti-NG2 (green). Yellow colour=vasculature-associated pericytes; green colour=pericytes-disassociated from the tumour vasculature. The right panels reflect magnification of the boxed regions in the middle panels ( × 20). Right: Quantification of microvasculature areas (top) ( n =7–9), pericyte numbers (middle) ( n =7), pericyte association (bottom) ( n =7) in T241-vector and -PDGF-BB tumours. ( d ) Left: LLC-vector and -PDGF-BB tumour tissues were immunostained as in a . Yellow colour=vasculature-associated pericytes; green colour=pericytes disassociated from the tumour vasculature. Right: Quantification of microvasculature areas (top) ( n =7–9), pericyte numbers (middle) ( n =7), pericyte association (bottom) ( n =7) in LLC-vector and -PDGF-BB tumours. ( e , f ) Top: T241-vector and -PDGF-BB ( c ) or LLC-vector and -PDGF-BB ( d ) tumour cells were mixed at different ratios and implanted in C57Bl/6 mice. The tumour vasculature and pericyte association were detected using anti-CD31 (red) and anti-NG2 (green) double immunostaining. Expression levels of PDGF-BB in tumours were analysed by ELISA. Yellow colour indicates vasculature-associated pericytes and green colour indicates pericytes disassociated from the vasculature. Arrows in e , f indicate the dilated and disorganized tumour vasculatures. Bottom: Quantification of pericyte numbers in vector and PDGF-BB tumours ( n =7) and pericyte association in control and PDGF-B tumour vasculatures ( n =7). All quantifications were performed using the × 20 magnification. Scale bar, 50 μm (in all images); V, vector tumours; P, PDGF-BB tumours. All data are repeated at least twice and represented as mean±s.e.m. * P <0.05; ** P <0.01; *** P <0.001 (Student’s t -test). Full size image PDGF-BB induces pericyte loss in mouse tumour models In mice implanted with T241 or LLC transfectants, the resulting PDGF-BB-expressing tumours contained a significantly higher density of CD31-positive vessels relative to controls ( Fig. 1c ). Surprisingly, NG2-positive pericytes were markedly reduced in PDGF-BB tumours compared with those lacking PDGF-BB expression ( Fig. 1c ). Residual NG2 + pericytes remained disassociated from blood vessels in PDGF-BB tumours ( Fig. 1c ) but were associated with blood vessels in PDGF-BB-negative tumours ( Fig. 1c ). Significant pericyte loss occurred in primary tumours that were relatively small, and pericytes were progressively lost during expansion of the tumour mass ( Supplementary Fig. S1 ). PDGF-BB induces dose-dependent pericyte loss To define levels of tumour-derived PDGF-BB in causing pericyte loss from tumour vessels, we designed an experiment in which various ratios of PDGF-BB and vector tumour cells were mixed to achieve gradient levels of PDGF-BB production in tumours. As expected, various ratios of mixtures between PDGF-BB and vector tumours created gradient concentrations of PDGF-BB production in both T241 and LLC tumour tissues ( Fig. 1e ). Intriguingly, in both tumour types, the total pericyte numbers were decreased starting from the concentration of ~13–32 pg PDGF-BB per mg tissue and progressively decreased at higher concentrations. Consistent with the loss of total pericyte numbers, most of the remaining pericytes were disassociated from the tumour vasculature ( Fig. 1e ). Moreover, the structure and architecture of tumour vessels became increasingly disorganized and tortuous along with elevated levels of PDGF-BB production, leading to the formation of primitive vascular plexuses. For example, at the concentration of ~1 ng mg −1 tissue, tumour microvessels appeared as enlarged vascular plexuses probably due to fusion or undirected growth of microvessels ( Fig. 1e arrows). Dose-dependent opposing vascular effects of anti-PDGFR-β PDGFR-β is the critical receptor expressed in pericytes involved in vascular remodelling under physiological and pathological conditions. To study the impact of PDGFR-β blockades on tumour vasculatures, T241-PDGF-BB and -vector tumours were treated with a neutralizing monoclonal antibody (2C5, 800 μg/mouse 2 × /week) specifically against mouse PDGFR-β (ref. 21 ) and imatinib, a potent tyrosine kinase inhibitor. Expectedly, treatment of T241-vector tumours with 2C5 and imatinib resulted in marked reduction of pericyte density and coverage ( Fig. 2a ). PDGFR-β blockades also significantly reduced tumour microvessel density relative to controls ( Fig. 2a ). Surprisingly, PDGFR-β blockades significantly increased the pericyte density and vascular coverage in T241-PDGF-BB tumours relative to untreated tumours although the total numbers of pericytes remained at a low level ( Fig. 2c ). Similar to T241-vector tumours ( Supplementary Fig. S2a,c ), treatment with PDGFR-β blockades led to a decreased vascular density and tumour growth in PDGF-BB tumours ( Fig. 2c and Supplementary Fig. S2b,e ). The opposing effects of PDGFR-β blockades on pericyte density and coverage in T241-PDGF-BB and -vector tumours were further validated using two sets of independent markers, endomucin and α-smooth muscle actin (α-SMA) that detect microvessels and pericytes/vascular smooth muscle cells (VSMCs) ( Supplementary Fig. S2c–f ). Notably, α-SMA staining also revealed a population of myofibroblasts in the stromal compartment ( Supplementary Fig. S2e ). 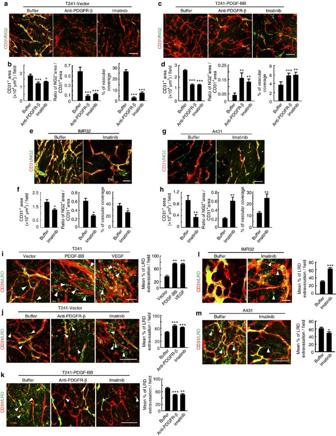Figure 2: Opposing effects of PDGFR-β blockade depend on tumour PDGF-BB production. (a,c) Representative images of T241-vector or -PDGF-BB tumour vasculatures (red) and pericytes (green) treated with buffer, anti-PDGFR-β antibody or imatinib. Yellow colour shows overlapping signals of red and green. (b,d) Left: Quantification of tumour microvascular density (n=8–10 fields per group). Middle: Quantification of the ratio of NG2+pericyte versus CD31+microvessels (n=8–10 fields per group). Right: Quantification of pericyte coverage in tumour vasculatures (n=8–10 fields per group). (e,g) Representative photos of IMR32 or A431 tumour vasculatures (red) and pericyte coverage (green) treated with buffer or imatinib. (f,h) Left: Quantification of microvascular areas in IMR32 (f) or A431 (h) tumours (n=9–11 fields per group). Middle: Quantification of the ratio of NG2+pericyte versus CD31+microvessels in IMR32 (f) or A431 (h) (n=9–11 fields per group). Right: Quantification of pericyte coverage in tumour vasculatures in IMR32 (f) or A431 (h) (n=9–11 fields per group). All scale bars, 50 μm. *P<0.05; **P<0.01; ***P<0.001 (Student’st-test). (i) Left: Vascular leakage of lysinated dextran (70 kDa) (green) and tumour vasculatures (red) in T241-vector, -PDGF-BB and -VEGF tumours were examined using a confocal microscope. Green=the extravasated dextran signals. Right: Quantification of percentages of extravasated dextran versus total dextran signals (n=10 randomized fields). (j,k) left: T241-vector or -PDGF-BB tumour vasculatures (red) and dextran (green) treated with buffer, anti-PDGFR-β antibody or imatinib. Green colour indicates the extravasated dextran. Right: Quantification of extravasated dextran in T241-vector tumours (j) (n=11–14 fields per group) or T241-PDGF-BB tumours (k) (n=7 fields per group). (l,m) Left: IMR32 or A431 tumour vasculatures (red) and dextran (green) treated with buffer or imatinib. Green colour indicates the extravasated dextran. Right: Quantification of extravasated dextran in IMR32 tumours (l) (n=13–15 fields per group) or A431 tumours (m) (n=15–21 fields per group). Scale bar, 50 μm (in all images). *P<0.05; **P<0.01; ***P<0.001 (Student’st-test). All data are repeated at least twice and represented as mean±s.e.m. Figure 2: Opposing effects of PDGFR-β blockade depend on tumour PDGF-BB production. ( a , c ) Representative images of T241-vector or -PDGF-BB tumour vasculatures (red) and pericytes (green) treated with buffer, anti-PDGFR-β antibody or imatinib. Yellow colour shows overlapping signals of red and green. ( b , d ) Left: Quantification of tumour microvascular density ( n =8–10 fields per group). Middle: Quantification of the ratio of NG2 + pericyte versus CD31 + microvessels ( n =8–10 fields per group). Right: Quantification of pericyte coverage in tumour vasculatures ( n =8–10 fields per group). ( e , g ) Representative photos of IMR32 or A431 tumour vasculatures (red) and pericyte coverage (green) treated with buffer or imatinib. ( f , h ) Left: Quantification of microvascular areas in IMR32 ( f ) or A431 ( h ) tumours ( n =9–11 fields per group). Middle: Quantification of the ratio of NG2 + pericyte versus CD31 + microvessels in IMR32 ( f ) or A431 ( h ) ( n =9–11 fields per group). Right: Quantification of pericyte coverage in tumour vasculatures in IMR32 ( f ) or A431 ( h ) ( n =9–11 fields per group). All scale bars, 50 μm. * P <0.05; ** P <0.01; *** P <0.001 (Student’s t -test). ( i ) Left: Vascular leakage of lysinated dextran (70 kDa) (green) and tumour vasculatures (red) in T241-vector, -PDGF-BB and -VEGF tumours were examined using a confocal microscope. Green=the extravasated dextran signals. Right: Quantification of percentages of extravasated dextran versus total dextran signals ( n =10 randomized fields). ( j , k ) left: T241-vector or -PDGF-BB tumour vasculatures (red) and dextran (green) treated with buffer, anti-PDGFR-β antibody or imatinib. Green colour indicates the extravasated dextran. Right: Quantification of extravasated dextran in T241-vector tumours ( j ) ( n =11–14 fields per group) or T241-PDGF-BB tumours ( k ) ( n =7 fields per group). ( l , m ) Left: IMR32 or A431 tumour vasculatures (red) and dextran (green) treated with buffer or imatinib. Green colour indicates the extravasated dextran. Right: Quantification of extravasated dextran in IMR32 tumours ( l ) ( n =13–15 fields per group) or A431 tumours ( m ) ( n =15–21 fields per group). Scale bar, 50 μm (in all images). * P <0.05; ** P <0.01; *** P <0.001 (Student’s t -test). All data are repeated at least twice and represented as mean±s.e.m. Full size image To exclude the possibility that the opposing effect of PDGFR-β blockades on pericyte coverage only occurred in T241 fibrosarcoma, LLC-PDGF-BB and -vector tumours were also used. Similar to T241 tumour models, PDGFR-β blockades significantly reduced tumour growth, pericyte density, vascular coverage, and microvessel density in LLC-vector tumours ( Supplementary Fig. S3a,c,d ), whereas the opposite results with exceptions of the tumour growth rate and vessel density were found in LLC-PDGF-BB tumours ( Supplementary Fig. S3b,e,f ). These findings were further validated with endomucin and α-SMA staining ( Supplementary Fig. S3g–j ). Despite the notable difference of PDGFR-β blockades on pericyte density and coverage, primary tumour growth rates were significantly inhibited in both PDGF-BB-positive and negative tumours. These findings demonstrate that microvessel density might be a key determinant for controlling tumour growth ( Supplementary Figs S2a,b and S3a,b ). To translate these findings to clinical relevance, we analysed naturally high and low PDGF-BB-producing human tumours. Similar to mouse tumour models seen in T241 and LLC, opposing effects of PDGFR-β blockades on pericyte density and coverage were also found in A431 and IMR32 human tumours ( Fig. 2e–h and Supplementary Fig. S4c–f ). However, growth rates of both tumours were significantly inhibited by PDGFR-β blockades ( Supplementary Fig. S4a,b ). To further validate these findings, we performed the same experiments using an orthotopic LLC tumour model. Orthotopic PDGF-BB LLC tumours exhibited an accelerated tumour rate, pericyte loss and imatinib response ( Supplementary Fig. S5 ), which were virtually indistinguishable from those observed in xenograft tumour models. PDGF-BB-induced pericyte loss promotes vascular leakiness To determine the functional consequences of PDGF-BB-induced pericyte ablation, vascular leakage in control vector and PDGF-BB-expressing T241 tumours was compared using lysinated rhodamine-labelled dextran (LRD, 70 kDa) (ref. 22 ). Interestingly, the PDGF-BB-expressing tumour vasculature exhibited high permeability, leading to extravasation of LRD into the extravascular space ( Fig. 2i ). Similarly, increased extravasation of LRD was also observed in the same type of T241 tumour with elevated VEGF expression ( Fig. 2i ) [22] . At 15 min post-injection, more than 70% of the LRD was extravasated from tumour blood vessels in both PDGF-BB- and VEGF-expressing tumours ( Fig. 2i ). In contrast, a majority of the LRD molecules remained within the blood vessels of the vector- tumours, although not all tumour vessels exhibited blood perfusion ( Fig. 2i ). These findings demonstrated that PDGF-BB-induced pericyte ablation led to functional impairment of the tumour blood vessels owing to increased vascular leakage. Opposing effects of PDGFR-β blockades on vascular leakage The opposing effects of PDGFR-β blockades on pericyte numbers, recruitment and loss in high and low PDGF-BB-producing tumours suggested a possibility of alteration of vascular functions in the tumour environment. To test this possibility, we analysed vascular leakiness in tumours using 70 kDa LRD. In agreement with the opposing effects on pericyte coverage in tumour vessels, treatment with PDGFR-β blockades led to increased vascular leakiness in PDGF-BB-negative T241 tumours ( Fig. 2j ). Conversely, significantly decreased vascular leakage was detected in PDGFR-β blockade-treated PDGF-BB-expressing T241 tumours ( Fig. 2k ). Similar to mouse tumours, treatments of PDGF-BB high and low expressing human tumours resulted in similar opposing effects on vascular leakiness ( Fig. 2l ). To study if PDGF-BB is able to ablate PCs from established tumours, EGFP + (enhanced green fluorescent protein) PDGF-BB-producing or vector tumour cells were injected into established EGFP − wt tumours at the size of about 0.2 cm 3 . Similar to the de novo formation of PDGF-BB tumours, PCs in PDGF-BB-producing areas were substantially fewer and residual NG2 + PCs remained disassociated from tumour vessels ( Supplementary Fig. S6 ). These findings validate the fact that tumour cell-derived PDGF-BB induced marked PC loss from the tumour vasculature. It appears that PDGF-BB-induced percyte loss is independent from the VEGF-VEGFR signalling system because inhibition of VEGF by a VEGF specific blockade did not affect the PDGF-BB-induced pericyte loss ( Supplementary Fig. S7 ). Dual effects of imatinib on circulating tumour cells As pericytes are crucial for maintenance of vascular integrity, which is tightly linked with tumour cell dissemination from the primary site and cancer metastasis, we next measured the number of circulating tumour cells (CTCs) in imatinib-treated and non-treated tumour-bearing mice. Notably, treatment of PDGF-BB-negative T241 tumours with imatinib led to a significantly increased number of GFP + -CTCs ( Fig. 3a ). The number of CTCs was markedly increased in PDGF-BB-T241 tumour-bearing mice compared with vector-T241 tumour-bearing mice ( Fig. 3a ). Treatment of PDGF-BB-T241 tumour-bearing mice with imatinib significantly reduced the number of CTCs ( Fig. 3a ). These findings demonstrate that treatments of PDGF-BB-positive and -negative tumours with the same anti-cancer drug lead to an opposite consequence of tumour cell dissemination. 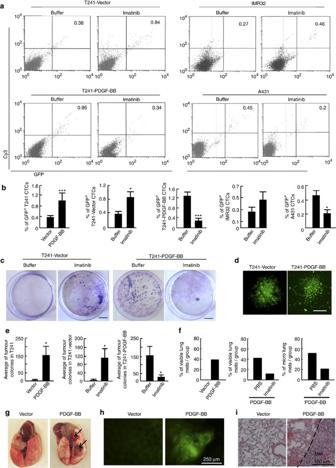Figure 3: Tumour PDGF-BB increases CTCs and pulmonary metastasis. (a) Left: Blood samples from T241-vector or -PDGF-BB tumour-bearing mice treated with or without imatinib were FACS analysed for EGFP+signals (right upper part of green fluorescent protein and Cy3 double-positive signals). Right: Blood samples from IMR32 or A431 tumour-bearing mice treated with or without imatinib were FACS analysed for EGFP+signals (right upper part on the each panel). (b) Quantifications of EGFP+signals in tumour-bearing mice blood with or without imatinib treatment (n=4–6 samples per group in T241,n=5 samples per group in IMR32 and A431, respectively). (c) Micrographs of representative cell culture dishes after incubation with blood samples from imatinib-treated or non-treated T241-vector or -PDGF-BB tumour-bearing mice. Blue colour indicates the Giemsa-positive tumour colonies. Scale bar, 2 cm. (d) Validation of EGFP+tumour colonies by fluorescent microscopy. Scale bar, 500 μm. (e) Quantification of tumour cell colonies in PB of T241-vector- and PDGF-BB tumour-bearing mice treated with or without imatinib (n=5–6 samples per group). All experiments were repeated at least two times. (f) Quantification of pulmonary metastasis in tumour bearing mice. Left: Quantification of visible metastatic lung nodules in T241-vector (n=10) or -PDGF-BB tumour (n=10) bearing mice. Middle: Quantification of visible metastatic lung nodules in T241-PDGF-BB tumour baring mice with (n=10) or without (n=10) imatinib. Right: Quantification of microscopic metastatic lung in T241-PDGF-BB tumour baring mice with (n=10) or without (n=10) imatinib. (g) Representative micrographs of lungs in T241-vector or -PDGF-BB tumour-bearing mice. Arrows indicate metastatic nodules. (h) EGFP+metastatic signals in the lung. Scale bar, 250 μm. (i) H&E staining in the lung of T241-vector or -PDGF-BB tumour-bearing mice. Met: metastatic lesion. Scale bar, 100 μm. All data except pulmonary metastasis are represented as mean±s.e.m. *P<0.05; ***P<0.001; (Student’st-test). All data are repeated at least twice. Figure 3: Tumour PDGF-BB increases CTCs and pulmonary metastasis. ( a ) Left: Blood samples from T241-vector or -PDGF-BB tumour-bearing mice treated with or without imatinib were FACS analysed for EGFP + signals (right upper part of green fluorescent protein and Cy3 double-positive signals). Right: Blood samples from IMR32 or A431 tumour-bearing mice treated with or without imatinib were FACS analysed for EGFP + signals (right upper part on the each panel). ( b ) Quantifications of EGFP + signals in tumour-bearing mice blood with or without imatinib treatment ( n =4–6 samples per group in T241, n =5 samples per group in IMR32 and A431, respectively). ( c ) Micrographs of representative cell culture dishes after incubation with blood samples from imatinib-treated or non-treated T241-vector or -PDGF-BB tumour-bearing mice. Blue colour indicates the Giemsa-positive tumour colonies. Scale bar, 2 cm. ( d ) Validation of EGFP + tumour colonies by fluorescent microscopy. Scale bar, 500 μm. ( e ) Quantification of tumour cell colonies in PB of T241-vector- and PDGF-BB tumour-bearing mice treated with or without imatinib ( n =5–6 samples per group). All experiments were repeated at least two times. ( f ) Quantification of pulmonary metastasis in tumour bearing mice. Left: Quantification of visible metastatic lung nodules in T241-vector ( n =10) or -PDGF-BB tumour ( n =10) bearing mice. Middle: Quantification of visible metastatic lung nodules in T241-PDGF-BB tumour baring mice with ( n =10) or without ( n =10) imatinib. Right: Quantification of microscopic metastatic lung in T241-PDGF-BB tumour baring mice with ( n =10) or without ( n =10) imatinib. ( g ) Representative micrographs of lungs in T241-vector or -PDGF-BB tumour-bearing mice. Arrows indicate metastatic nodules. ( h ) EGFP + metastatic signals in the lung. Scale bar, 250 μm. ( i ) H&E staining in the lung of T241-vector or -PDGF-BB tumour-bearing mice. Met: metastatic lesion. Scale bar, 100 μm. All data except pulmonary metastasis are represented as mean±s.e.m. * P <0.05; *** P <0.001; (Student’s t -test). All data are repeated at least twice. Full size image Consistent with mouse tumour models, treatment of natural PDGF-BB-expressing human A431 tumours with imatinib inhibited tumour cell dissemination, leading to a reduced total number of CTCs ( Fig. 3a ). Inversely, a trend of increased numbers of CTCs was found in PDGF-BB low-expressing IMR32 tumour-bearing mice ( Fig. 3a ). These data demonstrate that treatment of PDGF-BB-positive and -negative tumours with anti-PDGF agents can lead to opposing effects of tumour cell dissemination. To further study if the disseminated tumour cells are functionally relevant to cancer metastasis, we cultured the peripheral blood (PB) from tumour-bearing mice that were treated with or without imatinib. In concordance with CTC numbers, culturing of PB from T241-PDGF-BB tumour-bearing mice resulted in formation of a substantial number of tumour cell colonies ( Fig. 3c ), which were further validated by expression of EGFP ( Fig. 3d ). Conversely, only a few tumour cell colonies were detected in PB cultures from T241-vector tumour-bearing mice ( Fig. 3c ). However, treatment of PDGF-BB-negative vector tumour-bearing mice with imatinib led to a significant increase of tumour cell colonies ( Fig. 3c ). The opposite results were observed with T241-PDGF-BB tumours ( Fig. 3c ). These results show that imatinib is likely to promote tumour cell dissemination and metastasis in PDGF-BB-negative tumour-bearing animals although this possibility in cancer patients warrants further validation. PDGF-BB promotes pulmonary metastasis To further study the pathophysiological relevance of our findings, a mouse spontaneous metastatic model was employed. Subcutaneous implantation of PDGF-BB-T241 tumour cells in mice led to an increased number of pulmonary surface metastases relative to the control group ( Fig. 3f ). The increased number of lung metastatic nodules did not seem to the consequence of enhanced tumour growth rate in the PDGF-BB group as microscopic metastatic foci was also proportionally increased in the PDGF-BB tumour-bearing animals ( Fig. 3f ). Expectedly, imatinib significantly blocked both visible and microscopic metastases in the PDGF-BB tumour-bearing mice ( Fig. 3f ). These findings support the notion that PDGDF-BB promotes metastasis by facilitating tumour cell dissemination from the primary site owing to the altered vascular structure in the tumour microenvironment. Prolonged PDGF-BB treatment downregulates PDGFR-β We next devoted our efforts to gain mechanistic insights that underlie PDGF-BB-induced pericyte loss in the tumour vasculature. As PDGFR-β is essentially required for PDGF-BB-induced pericyte loss, activation of PDGFR-β was studied in PDGF-BB-stimulated and non-stimulated pericytes. As expected, PDGFR-β became markedly phosphorylated after 10 min PDGF-BB stimulation at the concentrations of 10 and 100 ng ml −1 , despite the fact that the total amount of PDGFR-β was decreased in a ligand dose-dependent manner ( Fig. 4a ). At 100 ng ml −1 , PDGF-BB substantially downregulated the expression level of the PDGFR-β that became barely detectable ( Fig. 4a ). Surprisingly, prolonged stimulation of pericytes with PDGF-BB led to almost total suppression of PDGFR-β activation ( Fig. 4a ). Consistent with short-time stimulation, the total amount of PDGFR-β was significantly downregulated ( Fig. 4a ). These findings demonstrate that persistent stimulation with PDGF-BB at high dosages lead to suppression rather than stimulation of PDGFR-β activation in pericytes. 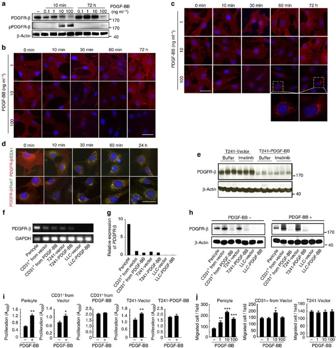Figure 4: PDGF-BB-induced downregulation of PDGFR-β and biological effects on non-pericytes. (a) Protein levels of total and the phosphorylated PDGFR-β (pPDGFR-β) in 0, 1, 10 or 100 ng ml−1PDGF-BB-treated pericytes. β-actin levels were used as standard loading. Non-permeabilized (b) and permeabilized (c) pericytes were stained with a specific anti-PDGFR-β antibody after stimulation with 1, 10 and 100 ng ml−1PDGF-BB for 0, 10, 30 and 60 min, and 72 h. Scale bar, 50 μm. (d) Permeabilized pericytes that were treated with 100 ng ml−1PDGF-BB for the indicated time points were double immunostained with a specific anti-PDGFR-β antibody (red) in combination with an early endosomal marker (EEA1) (green) or a later endosomal marker (Rab7) (green). Scale bar, 50 μm. (e) Total PDGFR-β protein expression levels were analysed in imatinib-treated or non-treated vector or PDGF-BB tumours. β-actin levels were used as standard loading controls. mRNA (f,g) and protein (h) expression levels of PDGFR-β in various cell types were detected by RT–PCR (f), by q-PCR (g) and by western blotting (h). GAPDH were used as standard loading controls for mRNA analysis and β-actin levels were used as standard loading controls for protein analysis. Proliferation (i) and migration (j) of various cell types in response to PDGF-BB stimulation were analysed (n=6–8). All data are repeated at least twice and represented as mean±s.e.m. *P<0.05; **P<0.01, ***P<0.001; (Student’st-test). All original gel pictures associated to this figure is shown inSupplementary Fig. S8. Figure 4: PDGF-BB-induced downregulation of PDGFR-β and biological effects on non-pericytes. ( a ) Protein levels of total and the phosphorylated PDGFR-β (pPDGFR-β) in 0, 1, 10 or 100 ng ml −1 PDGF-BB-treated pericytes. β-actin levels were used as standard loading. Non-permeabilized ( b ) and permeabilized ( c ) pericytes were stained with a specific anti-PDGFR-β antibody after stimulation with 1, 10 and 100 ng ml −1 PDGF-BB for 0, 10, 30 and 60 min, and 72 h. Scale bar, 50 μm. ( d ) Permeabilized pericytes that were treated with 100 ng ml −1 PDGF-BB for the indicated time points were double immunostained with a specific anti-PDGFR-β antibody (red) in combination with an early endosomal marker (EEA1) (green) or a later endosomal marker (Rab7) (green). Scale bar, 50 μm. ( e ) Total PDGFR-β protein expression levels were analysed in imatinib-treated or non-treated vector or PDGF-BB tumours. β-actin levels were used as standard loading controls. mRNA ( f , g ) and protein ( h ) expression levels of PDGFR-β in various cell types were detected by RT–PCR ( f ), by q-PCR ( g ) and by western blotting ( h ). GAPDH were used as standard loading controls for mRNA analysis and β-actin levels were used as standard loading controls for protein analysis. Proliferation ( i ) and migration ( j ) of various cell types in response to PDGF-BB stimulation were analysed ( n =6–8). All data are repeated at least twice and represented as mean±s.e.m. * P <0.05; ** P <0.01, *** P <0.001; (Student’s t -test). All original gel pictures associated to this figure is shown in Supplementary Fig. S8 . Full size image To further study the PDGF-BB-triggered suppression of PDGFR-β expression, cell surface PDGFR-β molecules were kinetically immunostained at various time points. Prolonged stimulation of pericytes with PDGF-BB resulted in marked decreased levels of cell surface PDGFR-β expression, which was virtually undetectable after 60 min stimulation at 100 ng ml −1 ( Fig. 4b ). Interestingly, an intracellular punctuated staining pattern of PDGFR-β signals were detected in prolonged PDGF-BB-stimulated pericytes ( Fig. 4c ), suggesting PDGF-BB-triggered internalization of PDGFR-β. Receptor internalization usually involves in endocytosis. Co-localization of PDGFR-β molecules with an early endosomal marker, early endosome antigen 1, and a late endosomal marker, Ras-related protein Rab-7 (Rab7), showed kinetic accumulation of PDGFR-β molecules in early endosomes, followed by late endosomes ( Fig. 4d ). These findings demonstrate that cell surface internalization of PDGFR-β molecules is a mechanism that underlies PDGF-BB-induced downregulation of PDGFR-β. Consistent with these in vitro findings, PDGFR-β expression levels were markedly downregulated in PDGF-BB tumour tissues and imatinib treatment did not significantly alter expression levels ( Fig. 4e ). Endothelial and tumour cell PDGFR-β and PDGF-BB effects As PDGF-BB is a pleiotropic factor that acts on several cell types in the tumour microenvironment, we analysed expression levels of PDGFR-β in non-pericyte cell types including tumour cells and ECs. The fibroblast-origin T241 fibrosarcoma cells expressed PDGFR-β mRNA and protein ( Fig. 4f–h ). In contrast, the epithelium-origin LLC tumour cells completely lacked PDGFR-β expression. Similar to T241 tumour cells, ECs isolated from the vector-tumour tissues also express PDGFR-β mRNA and protein ( Fig. 4f–h ). Interestingly, both ECs isolated from PDGF-BB tumours and PDGF-BB tumour cells expressed significantly lower or barely detectable levels of PDGFR-β mRNA and protein, suggesting that persistent expression of PDGF-BB in the tumour microenvironment led to downregulation of PDGFR-β in ECs and tumour cells as seen in pericytes. Consistent with PDGFR-β expression, stimulation of ECs and T241 cells with PDGF-BB resulted in proliferative or migratory activity ( Fig. 4i ), indicating that PDGF-BB in the tumour microenvironment might target other cell types other than pericytes. It is noteworthy to mention that the biological effect of PDGF-BB on ECs and tumour cells was virtually completely abolished in PDGF-BB tumours owing to downregulation of PDGFR-β expression by persistent PDGF-BB exposure ( Fig. 4f–h ). PDGFR-β-dependent regulation of integrin α1β1 by PDGF-BB We carried out a genome-wide gene expression analysis in PDGF-BB-stimulated and -non-stimulated pericytes. We were particularly interested in cell adhesion molecules that are involved in EC-pericyte interaction and attachment, and therefore collected all genes differentially expressed (false-discovery rate (FDR) <0.05) upon PDGF-BB treatment. These genes were annotated to ‘adhesion’ by the gene ontology consortium. Intriguingly, expression levels of signalling molecules involved in cell adhesion functions seemed to be markedly downregulated by PDGF-BB stimulation ( Fig. 5 ). Among all cell adhesion molecules, integrin α1 is the most downregulated adhesion molecule (>5-fold downregulation) in PDGF-BB-stimulated pericytes ( Fig. 5a ). Comparative analysis of all integrins confirmed the fact that integrin α1 was the most altered integrin molecule upon PDGF-BB stimulation ( Fig. 5b ). The genome-wide microarray analysis was further validated using a quantitative real-time PCR approach ( Fig. 5c ). After 24 h PDGF-BB stimulation at 100 ng ml −1 , nearly 30-fold downregulation of integrin α1 was detected in PDGF-BB-stimulated pericytes relative to the non-treated cells ( Fig. 5c ). 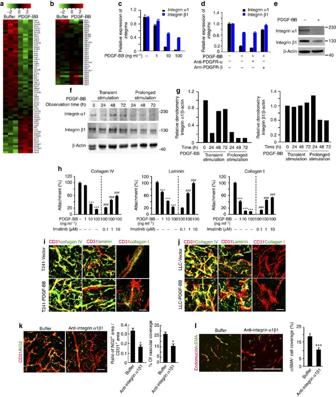Figure 5: Inactivation of PDGFR-β-mediated downregulation of integrin α1β1 leads to pericyte loss. (a,b) Affymetrix gene-array analysis on PDGF-BB- or buffer-treated pericytes for 5 days (n=3 per group). Heatmaps of the magnitude of differential expression (log2 scale) of adhesion-associated genes. (c) Relative fold induction ofintegrinα1orintegrinβ1mRNA with or without PDGF-BB (n=4). (d) Relative fold induction ofintegrinα1orintegrinβ1mRNA by PDGF-BB in the absence (control) or presence of antibodies against PDGFR-α or PDGFR-β (n=4). (e) Detection of integrin α1 and integrin β1 protein levels in PDGF-BB-treated or non-treated pericytes for 72 h. (f,g) Integrin α1 and integrin β1 protein levels upon transient (10 min) and prolonged stimulation with PDGF-BB. β-actin levels were used as standard loading controls. (h) Adhesion of pericytes to collagen IV, laminin or collagen I. Pericytes were pre-incubated with or without various concentrations of imatinib for 4 h, followed by treatment with PDGF-BB for 72 h. Values are shown as percentage changes (n=4). ***P<0.001;###P<0.001; Student’st-test. *Indicates significant difference between the non-treated pericytes and PDGF-BB-treated pericytes without imatinib.#Indicates significant difference between PDGF-BB-treated pericytes in the presence or absence of imatinib. (i) Representative images of T241-vector or -PDGF-BB tumour vasculatures (red) and collagen IV (green, left panel), laminin (green, middle panel) or collagen I (green, right panel). (j) Representative images of LLC-vector or -PDGF-BB tumour vasculatures (red) and collagen IV (green, left panel), laminin (green, middle panel) or collagen I (green, right panel). (k) Left: Representative images of T241-vector vasculature (red) and pericytes (green) treated with buffer or an anti-integrin α1β1 neutralizing antibody. Middle and right panels: Quantification of the ratio of NG2+pericytes versus CD31+microvessels (n=7 fields per group) and pericyte coverage in tumour vasculatures (n=7 fields per group). *P<0.05; Student’st-test. (i) Left: T241-vector tumour vessel treated with buffer or anti-integrin α1 antibody were detected by double immunostaining with endomucin (red) and αSMA (green) (n=12 fields per group). Scale bar, 50 μm (i,j,k) or 100 μm (l) (in all images). All experiments are repeated at least twice and represented as mean±s.e.m. ***P<0.001; (Student’st-test). All original gel pictures associated to this figure is shown inSupplementary Fig. S8. Figure 5: Inactivation of PDGFR-β-mediated downregulation of integrin α1β1 leads to pericyte loss. ( a , b ) Affymetrix gene-array analysis on PDGF-BB- or buffer-treated pericytes for 5 days ( n =3 per group). Heatmaps of the magnitude of differential expression (log2 scale) of adhesion-associated genes. ( c ) Relative fold induction of integrin α 1 or integrin β 1 mRNA with or without PDGF-BB ( n =4). ( d ) Relative fold induction of integrin α 1 or integrin β 1 mRNA by PDGF-BB in the absence (control) or presence of antibodies against PDGFR-α or PDGFR-β ( n =4). ( e ) Detection of integrin α1 and integrin β1 protein levels in PDGF-BB-treated or non-treated pericytes for 72 h. ( f , g ) Integrin α1 and integrin β1 protein levels upon transient (10 min) and prolonged stimulation with PDGF-BB. β-actin levels were used as standard loading controls. ( h ) Adhesion of pericytes to collagen IV, laminin or collagen I. Pericytes were pre-incubated with or without various concentrations of imatinib for 4 h, followed by treatment with PDGF-BB for 72 h. Values are shown as percentage changes ( n =4). *** P <0.001; ### P <0.001; Student’s t -test. *Indicates significant difference between the non-treated pericytes and PDGF-BB-treated pericytes without imatinib. # Indicates significant difference between PDGF-BB-treated pericytes in the presence or absence of imatinib. ( i ) Representative images of T241-vector or -PDGF-BB tumour vasculatures (red) and collagen IV (green, left panel), laminin (green, middle panel) or collagen I (green, right panel). ( j ) Representative images of LLC-vector or -PDGF-BB tumour vasculatures (red) and collagen IV (green, left panel), laminin (green, middle panel) or collagen I (green, right panel). ( k ) Left: Representative images of T241-vector vasculature (red) and pericytes (green) treated with buffer or an anti-integrin α1β1 neutralizing antibody. Middle and right panels: Quantification of the ratio of NG2 + pericytes versus CD31 + microvessels ( n =7 fields per group) and pericyte coverage in tumour vasculatures ( n =7 fields per group). * P <0.05; Student’s t -test. ( i ) Left: T241-vector tumour vessel treated with buffer or anti-integrin α1 antibody were detected by double immunostaining with endomucin (red) and αSMA (green) ( n =12 fields per group). Scale bar, 50 μm ( i , j , k ) or 100 μm ( l ) (in all images). All experiments are repeated at least twice and represented as mean±s.e.m. *** P <0.001; (Student’s t -test). All original gel pictures associated to this figure is shown in Supplementary Fig. S8 . Full size image The marked downregulation of integrin α1 by PDGF-BB promoted us to further study the role of integrin α1 in modulation of pericyte coverage in tumour vessels. Functional integrins require assembly of various combinations of alpha-chains with beta chains. As integrin α1 can only form the heterodimer with integrin β1 (refs 23 , 24 ), we also analysed the expression level of integrin β1 in PDGF-BB-stimulated pericytes. Interestingly, integrin β1 is also significantly downregulated by PDGF-BB in pericytes (>2-fold downregulation; Fig. 5c ). To further validate these findings at the protein level, we performed western immunoblotting using specific integrin α1 and integrin β1 antibodies. Expectedly, integrin α1 and integrin β1 protein levels were also markedly downregualted in PDGF-BB-treated pericytes ( Fig. 5f ). We next studied the involvement of PDGFR-α and PDGFR-β in mediating the PDGF-BB-induced downregulation of integrin α1 and integrin β1. Interestingly, the PDGFR-β blockade, but not PDGFR-α blockade, nearly completely inhibited the PDGF-BB-induced downregulation of integrin α1 and integrin β1 in pericytes ( Fig. 5d ). These findings demonstrate that cell adhesion molecules, integrin α1 and integrin β1, are markedly downregulated through the PDGF-BB-PDGFR-β-signalling system. Downregulation of integrin α1 could potentially be a downstream consequence of the PDGF-BB-triggered PDGFR-β repression. If this is the case, PDGFR-β-mediated signalling should positively upregulate integrin α1 expression. Indeed, transient stimulation of pericytes with PDGF-BB resulted in significant upregulation of integrin α1 expression ( Fig. 5f ). However, prolonged stimulation with PDGF-BB resulted in marked decrease of integrin α1 levels ( Fig. 5f ), reconciling with PDGF-BB-triggered inactivation of the PDGFR-β signalling. Similarly, prolonged PDGF-BB stimulation also resulted in downregulation of integrin β1 expression ( Fig. 5f ). Involvement of integrin α1β1-binding matrix proteins Integrin α1β1 binds to extracellular matrix proteins collagen I, IV and laminin. In the in vitro experiments, pericytes attached to these integrin α1β1-binding ligands, which were inhibited by PDGF-BB in a dose-dependent manner ( Fig. 5h ). Imatinib treatment largely restored the pericyte attachment to these matrix proteins ( Fig. 5h ). We next localized expression of α1β1 ligands, collagen I, IV and laminin in tumours in relation to the tumour vasculature. Interestingly, collagen IV, but not collagen I and laminin, is expressed in tumour microvessels ( Fig. 5i ). These findings reconcile with previous reports that collagen IV is one of the components of vascular associated matrix [25] . To further study the involvement of integrin α1β1 in pericyte association with tumour vessels, we treated T241 tumours with an anti-mouse integrin α1β1 neutralizing antibody [26] to reproduce PDGF-BB-induced pericyte loss. If integrin α1β1 mediates PDGF-BB-induced pericyte loss, treatment of tumours with the anti-mouse integrin α1β1 neutralizing antibody should produce a similar effect of pericyte loss in the tumour vasculature. Indeed, treatment of T241 tumours with the anti-mouse integrin α1β1 neutralizing antibody led to significant loss of pericytes and vascular coverage ( Fig. 5k ). These findings were further validated using independent markers including endomucin and α-SMA staining ( Fig. 5l ). These findings show that inhibition of integrin α1β1 at least could in part reproduce the PDGF-BB-induced pericyte loss in tumour vessels. Several key issues regarding the role of pericytes in tumour angiogenesis and antiangiogenic therapy need to be resolved. These include (1) would high numbers of pericytes be advantageous for tumour growth and metastasis? (2) If so, what is the relation of vascular pericyte coverage to tumour growth and metastasis? (3) Would the expression levels of PDGF-BB in various tumours be the key determinants of pericyte numbers and vascular coverage? (4) Would the cellular source of PDGF-BB be crucial for vascular pericyte coverage? (5) In PDGF-BB non- or low expressing tumours, would the anti-PDGF drugs produce beneficial effects for cancer patients? Or, would these drugs be harmful to cancer patients by promoting cancer progression and metastasis? (6) What would be the optimal surrogate marker for patient selection to maximize clinical benefits? In the present study, we provide compelling evidence to address some of these clinically relevant questions using mouse and human tumour models. Ablation of pericytes by anti-PDGF agents has been reported to increase vascular tortuosity and tumour growth, suggesting that anti-PDGF-BB-induced pericyte loss has a negative role in tumour angiogenesis and growth [3] , [27] . In contrast to these findings, PDGF-BB-induced vascular remodelling via recruitment of pericytes to angiogenic vessels has been proposed to normalize the disorganized and leaky tumour vasculature [20] , [28] . The controversial views of PDGF-pericytes in tumour angiogenesis and drug responses described by various groups may simply reflect the fact that tumours express different levels of PDGF-BB. As PDGF-BB is a potent chemotactic factor for targeted cells, which include VSMCs and pericytes; tumour cell-derived PDGF-BB may attract pericytes away from angiogenic vessels, leading to decreased coverage and eventually completely loss of pericytes ( Fig. 6 ). In a gradient PDGF-BB expression experiment using two independent tumour types, we demonstrated that PDGF-BB-induced pericyte detachment was observed at a concentration about 13–32 pg ml −1 , which is clinically relevant. Analyses of a range of human cell lines originated from different types of tumour tissues show that a broad range of expression levels of PDGF-BB exist in human tumours. Similar to mouse tumours, expression of PDGF-BB above this level in human tumours leads to decreased pericyte numbers, vascular coverage and tortuosity. Conversely, those human tumours under the threshold level generally exhibit a broad spectrum of pericyte coverage in angiogenic vessels. Based on these findings, we reasonably propose that PDGF-BB secreted from tumour cells establishes an extravascular PDGF-BB gradient that draws pericytes away from the surface of blood vessels ( Fig. 6 ). Thus, high levels of tumour cell-derived PDGF-BB prevent pericyte recruitment to angiogenic vessels and, in effect, ablate those pericytes existing in the established vasculature. The structural and functional impacts of pericyte alterations on tumour vessels are reflected by high degrees of vascular tortuosity and vascular leakiness. 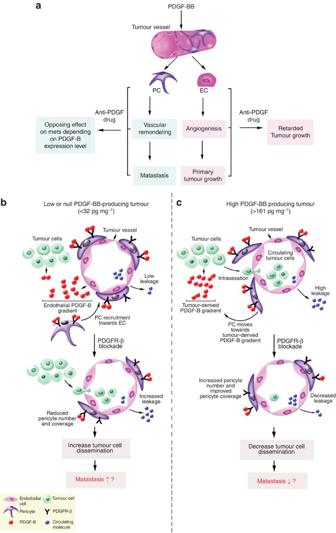Figure 6: Opposing effects of PDGFR-β blockades on metastasis. (a) PDGF-BB controls angiogenesis and vascular remodeling by targeting ECs and pericytes. Although modulation of angiogenesis directly participates in regulation of tumour growth, vascular remodeling is crucial for tumour cell dissemination in the circulation and subsequent metastasis. Our present data demonstrate that anti-PDGF agents suppress angiogenesis leading to retarded tumour growth in both low and high PDGF-expressing tumours. High levels of PFGF-B expressing tumours accelerate tumour cell dissemination and metastasis by inducing the formation of disorganized vascular networks lacking pericyte coverage. As a result, treatment of tumours with anti-PDGF-BB agents may lead to opposing effects on cancer metastasis depending on the expression levels of PDGF-BB. (b) In low or null PDGF-BB-producing tumours, vascular EC-derived PDGF-BB builds up a gradient that recruits pericytes through the PDGFR-β-signaling pathway onto the angiogenic vessels, leading to less leakiness. However, treatment of this type of tumour with PDGFR-β blockades blocks functions of EC-derived PDGF-BB, leading to reduced vascular pericyte coverage and increased vascular leakiness. The consequence of anti-PDGF-BB treatment in the tumour environment may manifest as increased tumour cell dissemination from the primary site and enhanced metastasis. (c) In high PDGF-BB-producing tumours (level >161 pg mg−1), tumour cell-derived PDGF-BB creates a gradient around tumour cells that attract pericytes away from the vasculature, leading to elevated levels of vascular leakage, which may provide structural basis of intravasation of tumour cells into the circulation and metastasis. PDGFR-β blockades could prevent the PDGF-BB-induced vascular leakiness and tumour cell dissemination. Thus, the same anti-PDGF-BB drug might have opposing effects on vascular leakage and tumour cell dissemination depending on the levels of PDGF-BB expression in tumours. Figure 6: Opposing effects of PDGFR-β blockades on metastasis. ( a ) PDGF-BB controls angiogenesis and vascular remodeling by targeting ECs and pericytes. Although modulation of angiogenesis directly participates in regulation of tumour growth, vascular remodeling is crucial for tumour cell dissemination in the circulation and subsequent metastasis. Our present data demonstrate that anti-PDGF agents suppress angiogenesis leading to retarded tumour growth in both low and high PDGF-expressing tumours. High levels of PFGF-B expressing tumours accelerate tumour cell dissemination and metastasis by inducing the formation of disorganized vascular networks lacking pericyte coverage. As a result, treatment of tumours with anti-PDGF-BB agents may lead to opposing effects on cancer metastasis depending on the expression levels of PDGF-BB. ( b ) In low or null PDGF-BB-producing tumours, vascular EC-derived PDGF-BB builds up a gradient that recruits pericytes through the PDGFR-β-signaling pathway onto the angiogenic vessels, leading to less leakiness. However, treatment of this type of tumour with PDGFR-β blockades blocks functions of EC-derived PDGF-BB, leading to reduced vascular pericyte coverage and increased vascular leakiness. The consequence of anti-PDGF-BB treatment in the tumour environment may manifest as increased tumour cell dissemination from the primary site and enhanced metastasis. ( c ) In high PDGF-BB-producing tumours (level >161 pg mg −1 ), tumour cell-derived PDGF-BB creates a gradient around tumour cells that attract pericytes away from the vasculature, leading to elevated levels of vascular leakage, which may provide structural basis of intravasation of tumour cells into the circulation and metastasis. PDGFR-β blockades could prevent the PDGF-BB-induced vascular leakiness and tumour cell dissemination. Thus, the same anti-PDGF-BB drug might have opposing effects on vascular leakage and tumour cell dissemination depending on the levels of PDGF-BB expression in tumours. Full size image The opposing vascular effects of high and low PDGF-BB levels in the tumour environment raise an important issue of clinical responses to drugs that target the PDGF pathways. Although drugs targeting the PDGF-signalling pathways are generally believed to be beneficial to cancer patients, in low PDGF-BB or non-producing tumours, these drugs likely block EC-derived PDGF-BB, leading to pericyte ablation, increased vascular tortuosity, and leakiness. In cancer patients, such drug-induced vascular changes may lead to increased levels of tumour cell dissemination and metastasis. In animal tumour models, we provide compelling evidence showing that treatment of PDGF-BB-negative tumours with PDGFR-β blockades resulted in increased populations of CTCs that form tumour spheroids in vitro . Although PDGFR-β blockades significantly inhibited neovascularization in PDGF-BB-expressing and non-expressing tumours, the same drug treatment leads to opposing effects on cancer metastasis. These findings provide convincing evidence that alteration of vascular structure rather than numbers is the key determinant for dissemination of tumour cells from the primary site ( Fig. 6 ). Pericytes have a crucial role in maintaining vascular integrity and stability. Ablation of pericytes by tumour-derived PDGF-BB alters the vascular structure toward disorganized premature vascular plexuses, leading to easy access of tumour cells into the circulation. Conversely, PDGF-BB-targeted EC proliferation or migration may be reflected in the tumour environment as increased neovascularization that results in an accelerated tumour growth rate. Based on our findings, we propose a mechanistic model in which PDGF-BB-induced EC-angiogenesis accelerates primary tumour growth, whereas PDGF-BB-targeted pericyte-vascular remodelling mediates metastasis ( Fig. 6 ). Another important and clinically relevant aspect from our present work is that expression levels of PDGF-BB in tumours might potentially serve as a surrogate marker to achieve personalized therapy. In patients with PDGF-BB-negative tumours, delivery of anti-PDGF drugs should proceed with great cautions as these agents might increase cancer spread. These findings need to be further validated in clinical settings. Taken together, our findings have shed new light on molecular mechanisms underlying clinical benefits of ongoing antiangiogenic therapy using anti-PDGF drugs such as imatinib and pave new avenues for further clinical practice of these important drugs by targeting the PDGF-signalling pathway. Animals See Supplementary Methods for details. All mouse studies were approved by the Northern Stockholm Experimental Animal Ethical Committee. Isolation of CD31 + cells from tumour tissues by FACS Subcutaneous vector- and PDGF-BB-T241 tumour tissues were prepared as single-cell suspensions, followed by incubation for 60 min at 37 °C with a solution containing 0.15% collagenase I and II. Cells were stained for 45 min on ice with a rat anti-mouse CD31 antibody (1:100; BD-Pharmingen, 553370). After rigorous washing with PBS, cells were incubated with an Alexa Fluor 555-labelled goat anti-rat antibody for 20 min on ice. CD31 + cells were analysed and sorted by FACS analysis as previously described [5] , [21] (MoFlo XTD, Beckman Coulter) and were cultured for further experimentation. Measurement of CTCs using FACS Xenograft tumour experiments were performed as previously described [22] , [29] , [30] , [31] , [32] . When tumour sizes in experimental (4–6 mice per group, 2–4 experiments) groups became equal, that is, 1.5 cm 3 , tumour-bearing mice were killed by a lethal dose of CO 2 . Fresh blood was intracardiacally collected from each mouse using a heparinized syringe immediately after mouse death. About 2.5 ml of red blood cell (RBC) lysis buffer (eBioscience, San Diego, CA) were added to 250 μl of fresh blood from each mouse and incubated. The lysis process was stopped by adding 10 ml PBS, followed by centrifugation at 1,500 r.p.m. for 5 min. The pellets were resuspended in 4% paraformaldehyde (PFA) and incubated for 15 min at room temperature. Cells were permeabilized using 0.15% Triton X-100 in PBS. Fixed and permeabilized cells were centrifuged at 1,500 r.p.m. for 5 min, followed by incubation with 2% bovine serum albumin in PBS to block non-specific binding sites. Cell pellets were washed and incubated on ice with a rabbit anti-EGFP antibody (1:50, Invitrogen AB, Sweden, A11122) for 45 min followed by goat anti-rabbit Cy3 (invitrogen AB, Sweden) incubation on ice for 30 min. Cell pellets were washed in PBS and replaced with 1% PFA in PBS. Samples were analysed by flow cytometry using FACScan and CellQuest software (BD, Franklin Lakes, NJ). Healthy mouse blood and EGFP + tumour sample alone was used for the control. Forward and side scatter gates were set and ~10,000 events were analysed per sample using CellQuest software. For analysis of human tumour cells, A431 and IMR32 cells were engineered to express EGFP using a lentiviral vector (GeneCopoeia Inc., Rockville, MD). Tumour colony formation Fresh blood samples were collected as mentioned above for FACS analysis and were subjected to DMEM supplemented with 10% FBS. The samples were incubated in 10 cm diameter cell culture dishes (Corning, NY) for 21 days. Tumour cell colonies were fixed 20 min with 4% PFA, followed by staining with Giemsa (Sigma). The stained tumour cell colonies were photographed using a digital camera (Canon, PC1089, Japan). Tumour colonies in the entire dish were counted using a Photoshop program (12–32 samples per group). EGFP signals of tumour colonies were detected using a fluorescence microscope equipped with a camera (Nikon, DS-QilMC). Whole-mount staining Immunohistochemical staining of whole-mount tissue samples was performed according to our previously published methods [33] , [34] , [35] , [36] , [37] , [38] . Treated and non-treated tumour tissues were fixed with 4% PFA overnight and cut into small pieces. Tissues were digested at room temperature with 20 mM proteinase K in 10 mM Tris buffer (pH 7.5) for 5 min, followed by incubation in 100% methanol for 30 min. Tissues were washed three times with PBS and incubated overnight at 4 °C in PBS containing 3% skim milk in 0.3% Triton X-100, followed by incubation with various combinations of a rat monoclonal anti-mouse CD31 (1:200; BD-Pharmingen, 553370), a rabbit polyclonal anti-NG2 (1:200; Millipore, AB5320), a rabbit anti-mouse collagen IV antibody (1:200; Abcam, ab19808), a rabbit anti-mouse laminin antibody (1:200; Abcam, ab30320) and a rabbit anti-mouse collagen I antibody (1:200; Abcam, ab21286). Anti-CD31 was used alone for LRD perfusion analysis. Samples were thoroughly rinsed, and blood vessel ECs and pericytes were detected using fluorescently labelled secondary antibodies of Alexa Fluor 555-labelled goat anti-rat (1:200; Invitrogen, A21434), Cy3-labelled goat anti-rabbit (1:200; Millipore, AP187C) and Cy5-labelled goat anti-rat (1:200; Millipore, AP183S). After washing, tissues were mounted using Vectashield mounting medium (Vector Laboratories, Burlingame, CA, USA) and were analysed by confocal microscopy (Zeiss Confocal LSM510 microscope; Carl Zeiss, Jena, Germany or Nikon C1 Confocal microscope, Nikon Corporation, Japan). Immunohistochemical staining Immunomhistochemical staining was performed according to previously published methods [39] , [40] , [41] . Paraffin-embedded tumour issue sections (5 μm) were double-stained with anti-endomucin (1:400; eBioscience, 14-5851-85) and anti-αSMA (1:200; DAKO, M0851) antibodies, followed by staining with a mixture of secondary antibodies comprised of Alexa Fluor 555-labelled goat anti-rat (1:400; Molecular Probes) and Alexa Fluor 488-labelled donkey anti-mouse (1:400; Molecular Probes). Positive signals were captured using a fluorescence microscope equipped with a camera (Nikon, DS-QilMC). Vascular permeability assay Tumour-bearing animals were anaesthetized by intraperitoneal injection of a mixture containing Hypnorm (fentanyl citrate and fluanisone; VetaPharma) and Dormicum (midazolam; Roche) [22] , [29] . Approximately 1.25 mg of lysinated LRD (70 kDa; Invitrogen, D1818) in 100 μl ddH 2 O was then intravenously injected into the tail vein of each animal. At 15 min post-injection, mice were killed by cervical dislocation and tumours were resected, followed by fixing in 4% PFA overnight. Whole-mount immunostaining of tumour tissues was performed with anti-CD31 followed by Cy5-labelled goat anti-rat IgG secondary antibody (1:200, Invitrogen, AP183S). Positive signals were examined by confocal microscopy. Pericyte adhesion assay Pericytes were pretreated with or without 1–100 ng ml −1 PDGF-BB for 72 h. A 48-well plate was coated with 50 ng ml −1 collagen I (Advanced BioMatrix, 5005-B), collagen IV (BD-Biosciences, 354233), or 15 ng ml −1 of laminin (BD-Biosciences, 354232) at 37 °C for 1 h, followed by incubation in a blocking buffer (2% bovine serum albumin in PBS) for 1 h. After washing three times, 1 × 10 4 cells in 100 ml were added to each well, followed by incubation for 20 min at 37 °C. Unattached cells were removed by rigorous washing. Adhesive cells were visualized and measured in a spectrophotometer at 405 nm wavelength by using the substrate, 4-nitrophenyl N -acetyl-β- D -glucosaminide (Sigma, N9376). Proliferation and migration assay Cell proliferation and migration assays were performed according to previously published methods [5] , [30] . Cell proliferation in the absence and presence of 100 ng ml −1 of rhPDGF-BB ( n =5) was analysed with MTT (Sigma) at 48 h after seeding into 96-well plates. Absorbance at 490 nm was detected by a spectrophotometer. Migrated cells stimulated by 0, 1, 10 and 100 ng ml −1 of rhPDGF-BB ( n =6) were examined using a Boyden chamber. Migrated cell numbers stained with Giemsa were photographed by light microscopy and counted using NIs-elements D1 software. Affymetrix gene-array analysis RNA samples were prepared using the RNAeasy (Qiagen) kit (control and PDGF-BB treatments after 5 days; three replicates for each condition) and were hybridized onto Affymetrix 1.0 ST Gene arrays. We used custom CDF definitions (ENTREZGENE) for data extraction [42] as these provide improved precision and accuracy [43] . Normalization was performed using robust multichip averaging (RMA) in R ( www.r-project.org ) by applying the ‘rma’ function within the ‘affy’ package (v1.32.1) and using default settings. Differentially expressed genes between each of the treated and untreated samples were identified using the random variance model two-tailed t -test. The resulting P -values were adjusted for multiple testing using the Benjamini–Hochberg FDR method [44] . Genes with an FDR <0.05 were considered differentially expressed. We used GO annotations to identify all differentially expressed genes that were also annotated to ‘adhesion’ and extracted data for all integrin genes. Per sample data for genes annotated to ‘adhesion’ and integrins were per gene normalized and ordered based on magnitude of differential expression. The data were displayed as heatmaps without applying hierarchical clustering. Gene-array data have been deposited in the Gene Expression Omnibus with an accession number GSE46564 . Statistical analysis Statistical analyses of in vitro and in vivo results were performed using the standard two-tailed Student t -test, and * P <0.05, ** P <0.01 and *** P <0.001 were considered statistically significant. Accession Codes Microarray data have been deposited in the Gene Expression Omnibus under accession code GSE46564 . How to cite this article: Hosaka, K. et al. Tumour PDGF-BB expression levels determine dual effects of anti-PDGF drugs on vascular remodelling and metastasis. Nat. Commun. 4:2129 doi: 10.1038/3129 (2013).